Photo-oxidative enhancement of polymeric molecular sieve membranes High-performance membranes are attractive for molecular-level separations in industrial-scale chemical, energy and environmental processes. The next-generation membranes for these processes are based on molecular sieving materials to simultaneously achieve high throughput and selectivity. Membranes made from polymeric molecular sieves such as polymers of intrinsic microporosity (pore size<2 nm) are especially interesting in being solution processable and highly permeable but currently have modest selectivity. Here we report photo-oxidative surface modification of membranes made of a polymer of intrinsic microporosity. The ultraviolet light field, localized to a near-surface domain, induces reactive ozone that collapses the microporous polymer framework. The rapid, near-surface densification results in asymmetric membranes with a superior selectivity in gas separation while maintaining an apparent permeability that is two orders of magnitude greater than commercially available polymeric membranes. The oxidative chain scission induced by ultraviolet irradiation also indicates the potential application of the polymer in photolithography technology. Membrane-separation technology has become a promising alternative to conventional energy-intensive separation processes such as distillation or absorption, for example, in natural gas sweetening, hydrogen recovery and production, carbon dioxide separation from flue gas and air separation [1] . State-of-the-art polymeric gas-separation membranes are subject to a trade-off between permeability and selectivity, as theoretically predicted by Freeman [2] , also known as the Robeson’s upper bound [3] , [4] . Research of the next-generation separation membrane is focused on tuning both local chemical interactions and pore sizes towards the kinetic diameter of molecules to achieve both selective separation and high throughput [1] , [5] , [6] , [7] , [8] , [9] , [10] , [11] , [12] , [13] , [14] . Over the past decade, significant progress has been made in molecular sieving materials such as carbon-based membranes (for example, carbon nanotubes [15] , [16] and graphene [9] ) and zeolites [7] . However, such membranes have not found commercial applications in gas separation because of high cost and scale-up impracticalities [17] . In contrast, microporous (pore sizes <2 nm) organic polymer materials are considered to have more impressive near-future impacts. Prospective classes of materials include metal-organic frameworks [18] , covalent organic frameworks [19] , substituted polyacetylenes, [20] thermally rearranged polymer [6] , conjugated microporous polymer [21] and polymers of intrinsic microporosity (PIMs) [10] , [11] , [12] , [22] , [23] , [24] , [25] . These microporous polymer materials have attracted significant interest for potential applications such as gas storage and separation, catalysis, energy storage and optoelectronics [26] . Among these microporous polymer materials, solution-processable PIMs have emerged as promising candidates of membrane materials for applications in large-scale gas separation [10] , [11] , [12] , [22] , [23] , [24] , [25] . A typical example is PIM-1 (see Supplementary Fig. S1 for structure and synthesis) [11] . The polymer repeating unit is rigidly kinked via a spiro-carbon centre that orthogonally connects two planar aromatic units. The kink leads to inefficient packing of polymer chains and a high fractional free volume. PIM class materials behave as molecular sieves (PIM-1 has a nominal pore size of<2 nm) and have extremely high gas permeability (for example, for PIM-1, permeability of CO 2 P CO2 ~5,000 Barrer, 1 Barrer=1 × 10 −10 cm 3 (STP)cm cm −2 s −1 cmHg −1 ) but only a moderate selectivity, α, which is defined as the relative permeability of one gas species to another. Hence, the selectivity of carbon dioxide over nitrogen and methane for PIM-1 are α CO2/N2 ~15–20 and α CO2/CH4 ~10, respectively, while the selectivity of oxygen over nitrogen is α O2/N2 ~3–4. In contrast, industrially used polymeric gas-separation membrane materials are much less permeable but achieve better selectivity (for example, for polyimide membranes, P CO2 is ~10 Barrer, and α CO2/CH4 is ~30). Currently, there are several strategies to improve the separation performance of PIMs membranes: (i) enhancing the rigidity of polymer chain by synthesis of new monomers [12] , [27] , [28] , [29] , [30] , (ii) post-synthetic modification of PIMs polymer [10] , [25] , [31] , (iii) mixed matrix membranes [32] , [33] , [34] and (iv) crosslinking induced by chemical [35] or heat treatment [36] . Ultraviolet light irradiation is a widely used technique for processing of polymer materials [8] , [37] , [38] , [39] , [40] , for example, polymerization of novel gas-separation membranes [40] , creating nanostructures from block copolymer [8] , or surface modification of polymeric films (for example, polyimides and polydimethylsiloxane) [8] , [37] , [38] , [39] . Enhancement of membrane-separation properties by ultraviolet surface modification is not uncommon. In fact, it has been used since the early start of polymer membrane-separation industry in the 1980s (ref. 41 ) [41] , for example, in crosslinking polyimide membranes containing benzophenone units [42] , [43] or degradation of siloxane-containing polymers [44] . However, the gas permeability of these conventional polymers is considerably low [45] . For the microporous PIMs polymers, understanding of the photo-oxidation phenomenon and stability is of broad interest to their wide range of applications (for example, gas separation, catalysis, optoelectronics and sensor). In this study, using PIM-1 as a prototype of microporous polymers, we demonstrate that oxidative chain scission of PIM-1 polymer occurs upon short-wavelength ultraviolet irradiation in the presence of oxygen. Owing to the limited penetration of ultraviolet light and ozone, the oxidative chain scission is restricted to the surface and led to a novel near-surface collapse and densification, which is especially pronounced in such open microporous polymeric materials. The resulting asymmetric membranes exhibit a superior selectivity in gas separation while maintaining an apparent permeability that is two orders of magnitude greater than commercially available polymeric membranes. The rapid transformation of the near-surface physical and chemical properties via this photo-oxidative technique suggests further applications in other thin-film technologies. Photo-oxidation and characterization of polymer films The ultraviolet irradiation ( λ =254 nm) of PIM-1 membranes in the presence of oxygen resulted in the asymmetric changes of membrane morphology. Cross-sectional scanning electron microscopy (SEM) image ( Fig. 1a ) shows the post-ultraviolet asymmetric physical changes at the surface of a 50-μm-thick membrane where a dense skin layer was formed above a more mesoporous intermediate layer (pore size about 2–20 nm, thickness about 0.1–2 μm). This intermediate layer was formed owing to the strain induced from densification of the skin layer; the remainder of the film was pristine PIM-1. The dense skin layer ( Fig. 1b ), forming quickly to a thickness of 300 nm within 10 min of ultraviolet exposure, thickened to 400 nm at longer exposure time (up to 60 min) ( Supplementary Figs S2 and S3 ). An identical trend was observed in 1.2-μm-thin films ( Fig. 1c ). 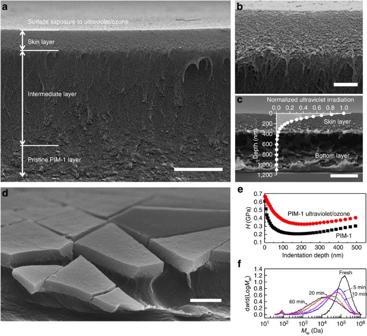Figure 1: Photo-oxidation of PIM-1 membranes. (a) Cross-sectional SEM of polymer of intrinsic microporosity (PIM-1) membrane (~50 μm thickness) after exposure to ultraviolet irradiation in air for 60 min, showing the formation of composite layers consisting of a denser skin layer and an intermediate mesoporous layer over the pristine dense PIM-1 layer. (b) Enlargement of cross-sectional SEM of surface layer. (c) Cross-sectional SEM of ultraviolet/ozone treated PIM-1 thin film. Inset shows the profile of ultraviolet light transmission as a function of depth. (d) Cross-sectional SEM of a fractured ultraviolet/ozone-treated PIM-1 membrane. Scale bar, 1 μm (ina,d); 200 nm (inb); 500 nm (inc). (e) Harness (H) as a function of indentation depth of pristine and ultraviolet/ozone-treated PIM-1 film. (f) Evolution of molecular weight distribution of PIM-1 thin film (~300 nm) exposure to ultraviolet irradiation in constant flow of pure O2(100 ml min−1) at different time. Figure 1c includes a superimposed plot of the transmitted intensity of ultraviolet light, I ( x ), through the depth, x , of the film. Described by a Beer–Lambert expression as I ( x )= I 0 exp(− x / L 0 ), the transmitted intensity decreased significantly from 8 mW cm −2 to 40 μW cm −2 at the depth of 500 nm, reflecting a characteristic penetration depth ( L 0 ) of ~105 nm for fresh PIM-1. This large attenuation in intensity comes from the fluorescent nature of PIM-1, which has an initial photoluminescence quantum yield efficiency of 37% ( Supplementary Fig. S4 ). The resulting surface-localized high ultraviolet field is responsible for much of the significant structural changes reported here. Figure 1: Photo-oxidation of PIM-1 membranes. ( a ) Cross-sectional SEM of polymer of intrinsic microporosity (PIM-1) membrane (~50 μm thickness) after exposure to ultraviolet irradiation in air for 60 min, showing the formation of composite layers consisting of a denser skin layer and an intermediate mesoporous layer over the pristine dense PIM-1 layer. ( b ) Enlargement of cross-sectional SEM of surface layer. ( c ) Cross-sectional SEM of ultraviolet/ozone treated PIM-1 thin film. Inset shows the profile of ultraviolet light transmission as a function of depth. ( d ) Cross-sectional SEM of a fractured ultraviolet/ozone-treated PIM-1 membrane. Scale bar, 1 μm (in a , d ); 200 nm (in b ); 500 nm (in c ). ( e ) Harness ( H ) as a function of indentation depth of pristine and ultraviolet/ozone-treated PIM-1 film. ( f ) Evolution of molecular weight distribution of PIM-1 thin film (~300 nm) exposure to ultraviolet irradiation in constant flow of pure O 2 (100 ml min −1 ) at different time. Full size image Mechanical properties During preparation of cross-sectional samples, very occasionally poorly fractured edges ( Fig. 1d ) indicated the contrast in mechanical properties of the skin and pristine regions. Nanoindentation measurements of the elastic modulus ( E ) and the hardness ( H ) were obtained on membranes at different conditions of ultraviolet irradiation using a sharp Berkovich tip in the continuous stiffness measurement mode ( Supplementary Fig. S5 and Supplementary Table S1 ). The representative hardness profiles with depth of membranes (0–500 nm) are shown in Fig. 1e . The pristine PIM-1 film with thickness of ~1 μm gave the overall Young’s modulus of ~6.94 GPa and hardness of ~0.23 GPa. After ultraviolet irradiation for 60 min in air, we found ~35% and ~50% increases of both Young’s modulus (9.00–9.33 GPa) and hardness (0.34–0.35 GPa), respectively. Equally it was found, from helium pycnometric studies, that the average density of the skin layer was 11% higher than the pristine PIM-1 film ( Supplementary Methods ). Molecular weight distribution Post-ultraviolet-treated membranes (50 μm thick) and thin films (100–1,000 nm) remained soluble in solvents (for example, chloroform or tetrahydrofuran), confirming that ultraviolet treatment did not result in crosslinking of polymer. Instead, gel permeation chromatography (GPC) measurements with PIM-1 thin film (~300 nm) showed that the average molecular weight decreased significantly. The pristine PIM-1 polymer has an average molecular weight of M n =100 kDa with a polydispersity index (PDI= M w / M n ) of 1.8. After ultraviolet irradiation in the presence of oxygen, the mean molecular weight decreases sharply indicating a broad range of fragmented polymer chains ( Fig. 1f ). However, the high PDI (~20) of the irradiated material limits the accuracy of characterizing the material with a single average molecular weight. This is to be expected from the attenuated ultraviolet light transmission with the depth of the thin film ( Fig. 1c ). The general observation of chain fragmentation was seen when samples were irradiated in air directly or through quartz glass ( Supplementary Fig. S6 ). These degraded fractions also became soluble in polar solvents (for example, dimethylformamide (DMF), acetone or methanol). In principle, such degradation can limit the gas-separation applications of such ultraviolet/ozone-modified PIM-1 films in environments with extended exposure to condensable organic vapours. However, we expect that further post-treatment of this selective surface layer can stabilize it against chemical erosion. Proposed mechanism of photo-oxidation It is well known that under short-wavelength ultraviolet irradiation, O 2 can absorb photons generating strongly oxidizing singlet oxygen and ozone. Equally, the high free volume and permeability of PIM-1 should lead to a local abundance of O 2 . Therefore, the PIMs materials behave as nanoreactors that are attacked by the oxidants generated within them, especially in the region of shallowly penetrating ultraviolet irradiation. We performed control experiments on ultraviolet irradiation of PIM-1 films in air, with films sandwiched between quartz glasses, which limited extent of oxygen exposure at the interface and carried out extensive characterization analyses. The conclusion of photo-oxidation and chain scission was essentially the same as those tests performed in air, or under gas flow with varied O 2 concentration. Oxidative chain scission occurred as schematically shown in Fig. 2a . The oxidation is supported by Fourier Transform infrared spectroscopy analysis indicating formation of carbonyl and hydroxyl groups in ultraviolet/ozone-treated samples ( Supplementary Fig. S7 ). Currently, the initial reaction site is still not clear and merits further study. The fragmented polymer segments pack more efficiently leading to loss of accessible free volume. This assumption was explored in molecular simulations of both PIM-1 ( Fig. 2b ) and the fragmented polymer ( Fig. 2c ). The accessible free volume, as probed by CO 2 molecules with a kinetic diameter of 3.3 Å at 298 K, was diminished in the simulation of densely packed shorter polymer chains. 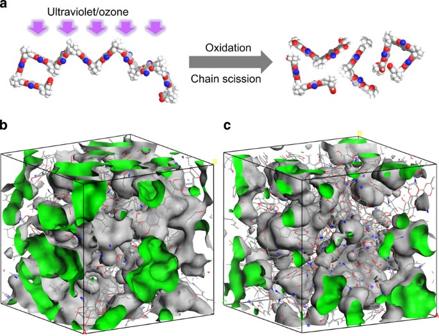Figure 2: Molecular structural transformation and simulation. (a) Schematic illustration of oxidative chain scission of PIM-1 upon exposure to ultraviolet irradiation in the presence of O2, showing transformation of long contorted polymer chains to shorter chains after oxidation and scission. (b) Three-dimensional view of computer simulation of an amorphous cell with PIM-1 polymer chains (four polymer chains inside, each containing of ten repeating units). Cell size: 31.8 × 31.8 × 31.8 Å, density of ~1.1 g cm−3. (c) Three-dimensional view of computer simulation of an amorphous cell with fragmented PIM-1, 20 polymer chains with two repeating PIM-1 units with oxidized groups, to mimic the shorter polymer chains after oxidative chain scission. Cell size: 29.5 × 29.5 × 29.5 Å, density of ~1.3 g cm−3. The grey surface indicates the van der Walls surface and green surface is the Connolly surface with probe radius of 1.65 Å. Figure 2: Molecular structural transformation and simulation. ( a ) Schematic illustration of oxidative chain scission of PIM-1 upon exposure to ultraviolet irradiation in the presence of O 2 , showing transformation of long contorted polymer chains to shorter chains after oxidation and scission. ( b ) Three-dimensional view of computer simulation of an amorphous cell with PIM-1 polymer chains (four polymer chains inside, each containing of ten repeating units). Cell size: 31.8 × 31.8 × 31.8 Å, density of ~1.1 g cm −3 . ( c ) Three-dimensional view of computer simulation of an amorphous cell with fragmented PIM-1, 20 polymer chains with two repeating PIM-1 units with oxidized groups, to mimic the shorter polymer chains after oxidative chain scission. Cell size: 29.5 × 29.5 × 29.5 Å, density of ~1.3 g cm −3 . The grey surface indicates the van der Walls surface and green surface is the Connolly surface with probe radius of 1.65 Å. Full size image Gas sorption properties N 2 adsorption at 77 K was performed with pristine PIM-1 thin films (~300 nm) and modified films after exposure to ultraviolet irradiation in air for 20 min. As shown in Fig. 3a , both pristine PIM-1 thin film and ultraviolet/ozone-treated PIM-1 thin film exhibited high sorption at very low relative pressure, which is typical of microporous polymer. Both samples show broad distributions of pore size as derived from the non-local density functional theory (NLDFT) method ( Supplementary Fig. S8 ). However, the ultraviolet/ozone-treated sample shows reduced pore volume over the range of 0.6–0.7 nm. This loss of microporosity resulted in the decrease of BET surface area from 779 to 573 m 2 g −1 and the micropore volume drops from 0.136 to 0.105 cm 3 g −1 . Similarly, we also observed a slight loss of CO 2 solubility in the ultraviolet/ozone-treated PIM-1 films ( Fig. 3a ). 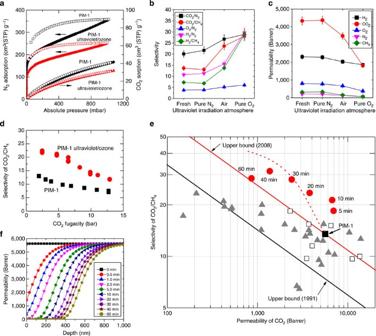Figure 3: Gas sorption and transport properties. (a) N2adsorption isotherms at 77 K and CO2sorption isotherms at 293 K. Ultraviolet/ozone-modified PIM-1 was prepared by ultraviolet irradiation of PIM-1 thin film (~300 nm) in air for 20 min. Solid and open symbols represent the adsorption and desorption branch, respectively. (b) Apparent selectivity and (c) gas permeability of pristine and ultraviolet-irradiated (20 min, 20 °C) PIM-1 membranes (~50 um) under different gas atmospheres. (d) Apparent selectivity of CO2/CH4of PIM-1 membrane (solid squares) and ultraviolet/ozone-treated (30 min) PIM-1 membrane (solid circles) as a function of fugacity of CO2in the mixed gas (CO2/CH4, 50/50 vol.%). (e) Apparent CO2/CH4selectivity versus apparent CO2permeability for PIM-1 (solid square) and ultraviolet/ozone-modified PIM-1 membranes (solid circles). The data are measured from pure-gas permeation tests with each gas repeated over three cycles of vacuum and permeation. The dashed line corresponds to model prediction. The dense membranes (~50 μm) were exposed to ultraviolet irradiation in air for varied time (5–60 min) as marked in the figure, with the membranes sandwiched in quartz glass. The open squares correspond to the literature data of PIM-1, the solid triangles represent the literature data of other PIMs, as summarized in a review by Duet al.46and data reported recently by Bezzuet al.30and Cartaet al.12The upper bounds were summarized by Robeson in 19913and 20084, respectively. (f) Prediction of transient intrinsic permeability of CO2along the depth of PIM-1 membrane upon exposure to ultraviolet irradiation. Figure 3: Gas sorption and transport properties. ( a ) N 2 adsorption isotherms at 77 K and CO 2 sorption isotherms at 293 K. Ultraviolet/ozone-modified PIM-1 was prepared by ultraviolet irradiation of PIM-1 thin film (~300 nm) in air for 20 min. Solid and open symbols represent the adsorption and desorption branch, respectively. ( b ) Apparent selectivity and ( c ) gas permeability of pristine and ultraviolet-irradiated (20 min, 20 °C) PIM-1 membranes (~50 um) under different gas atmospheres. ( d ) Apparent selectivity of CO 2 /CH 4 of PIM-1 membrane (solid squares) and ultraviolet/ozone-treated (30 min) PIM-1 membrane (solid circles) as a function of fugacity of CO 2 in the mixed gas (CO 2 /CH 4 , 50/50 vol.%). ( e ) Apparent CO 2 /CH 4 selectivity versus apparent CO 2 permeability for PIM-1 (solid square) and ultraviolet/ozone-modified PIM-1 membranes (solid circles). The data are measured from pure-gas permeation tests with each gas repeated over three cycles of vacuum and permeation. The dashed line corresponds to model prediction. The dense membranes (~50 μm) were exposed to ultraviolet irradiation in air for varied time (5–60 min) as marked in the figure, with the membranes sandwiched in quartz glass. The open squares correspond to the literature data of PIM-1, the solid triangles represent the literature data of other PIMs, as summarized in a review by Du et al . [46] and data reported recently by Bezzu et al . [30] and Carta et al . [12] The upper bounds were summarized by Robeson in 1991 [3] and 2008 [4] , respectively. ( f ) Prediction of transient intrinsic permeability of CO 2 along the depth of PIM-1 membrane upon exposure to ultraviolet irradiation. Full size image Gas transport properties We varied the concentration of O 2 in the ultraviolet irradiation atmosphere at a fixed exposure time (20 min) and found significant differences in pure gas permeation properties of PIM-1 membrane and ultraviolet/ozone-modified PIM-1, as shown in Fig. 3b–c . Pristine PIM-1 membrane presents a CO 2 permeability of ~4,500 Barrer, a CO 2 /N 2 selectivity of ~20 and a CO 2 /CH 4 selectivity at ~13, which are in agreement with the literature data [46] . Control experiments of ultraviolet exposure in pure N 2 showed no discernible difference in properties to that of pristine polymer. In contrast, increasing the concentration of O 2 (from 20.9 vol.% in air to pure O 2 ) enhanced the apparent selectivity of various gas pairs (for example, α CO2/N2 and α CO2/CH4 increased up to ~30) at the slight expense of permeability, corroborating the idea that ultraviolet-induced ozone within the open polymer network is responsible for subsequent structural densification. As practical applications of such membranes in separations involve mixtures of gases, the mixed gas selectivity of important gas pairs (such as CO 2 /CH 4 and CO 2 /N 2 ) was determined from equimolar gas mixtures indicating a significant enhancement in separation efficiency in ultraviolet-treated membrane (as seen for the CO 2 /CH 4 pair in Fig. 3d and also the CO 2 /N 2 gas pair in Supplementary Fig. S9 ). Moreover, these tests performed with clean cylinder mixed gas indicated the physical stability of the modified membranes at high pressure. We examined the dynamic change of gas transport properties of membranes exposed to ultraviolet irradiation in air for varied time of 5–60 min (for membranes exposed to air directly or membranes exposed to ultraviolet irradiation in air while sandwiched in quartz glass). Whether the membranes were exposed to air directly or sandwiched in quartz glass, we always observed the formation of densified skin layer ( Supplementary Fig. S3 ) and the decrease in molecular weight of the exposed PIM-1 ( Supplementary Fig. S6 ), confirming that the oxygen adsorbed within the polymer matrix was sufficient to induce the oxidation. However, sandwiching the membranes limited the source of O 2 at the interface and consequently slightly affected the reaction kinetics and resulting gas transport properties ( Supplementary Fig. S10 and Supplementary Table S2 ) without altering the general trend of lower permeability/higher selectivity for extended ultraviolet exposure. Here, we present the gas transport data of membranes exposed to ultraviolet irradiation in air, with the membranes sandwiched in quartz glass, as shown in Fig. 3e . Upon exposure to ultraviolet irradiation, the apparent permeability of CO 2 showed a slight increase (up to 7,000 Barrer) after short exposure for 5–10 min, but then decreased with extended exposure for 20–60 min, while the selectivity evidently increased. The slight increase of permeability after short exposure (5–10 min) of ultraviolet irradiation was within the error of measurement and subjected to plasticization and physical ageing during the history of measurement (multiple cycles of vacuum and permeation of several gases). It can effectively be considered a transient effect that becomes less significant when considered over the overall trends of permeability–selectivity performance in several sets of gas pair as shown later in Fig. 4 . The apparent selectivity of H 2 over each of N 2 and CH 4 increased up to ~60 with moderate decrease of permeability of H 2 (~2,000 Barrer). The apparent permeability of O 2 decreased to 600 Barrer with an O 2 /N 2 selectivity of ~6 ( Supplementary Table S2 and Supplementary Fig. S10 ). The overall membranes have apparent selectivity of commonly used gas-separation membrane materials while retaining orders-of-magnitude higher permeability. 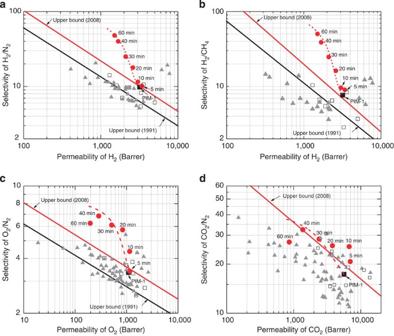Figure 4: Apparent gas transport properties. Apparent selectivity versus apparent permeability of PIM-1 and ultraviolet/ozone-modified PIM-1 membranes for industrially important gas pairs (a) H2/N2, (b) H2/CH4, (c) O2/N2and (d) CO2/N2. Solid squares: PIM-1 membrane; solid circles: ultraviolet/ozone-modified PIM-1 membranes; dashed lines: model predictions (seeSupplementary Note 1); solid lines: the upper bounds as summarized by Robeson in 19913and 20084, respectively; the open squares correspond to the literature data of PIM-1, the solid triangles represent the literature data of other PIMs, as summarized in a review by Duet al.46and data reported recently by Bezzuet al.30and Cartaet al.12The dense membranes (~50 μm) were exposed to ultraviolet irradiation in air for varied time (5–60 min) as marked in the figure, with the membranes sandwiched in quartz glass. The data are measured from pure-gas permeation tests at 4 bar at 22 °C. Figure 4: Apparent gas transport properties. Apparent selectivity versus apparent permeability of PIM-1 and ultraviolet/ozone-modified PIM-1 membranes for industrially important gas pairs ( a ) H 2 /N 2 , ( b ) H 2 /CH 4 , ( c ) O 2 /N 2 and ( d ) CO 2 /N 2 . Solid squares: PIM-1 membrane; solid circles: ultraviolet/ozone-modified PIM-1 membranes; dashed lines: model predictions (see Supplementary Note 1 ); solid lines: the upper bounds as summarized by Robeson in 1991 [3] and 2008 [4] , respectively; the open squares correspond to the literature data of PIM-1, the solid triangles represent the literature data of other PIMs, as summarized in a review by Du et al . [46] and data reported recently by Bezzu et al . [30] and Carta et al . [12] The dense membranes (~50 μm) were exposed to ultraviolet irradiation in air for varied time (5–60 min) as marked in the figure, with the membranes sandwiched in quartz glass. The data are measured from pure-gas permeation tests at 4 bar at 22 °C. Full size image The apparent gas transport properties of ultraviolet/ozone-modified membranes exceed the limitations defined by Robeson’s 2008 upper bound ( Fig. 3e ). However, it should be noted that as the membranes became asymmetric after modification, these measured permeability and selectivity are overall properties of the heterogeneous membrane. The Robeson’s upper-bound construction, on the other hand, reflects the intrinsic permeability and selectivity of homogeneous dense polymer membranes. Thus, in a strict sense, one should be careful to make a comparison of the performance of our ultraviolet/ozone-modified membranes to the upper bound. However, in a field where it is becoming more common to generate composite materials for gas separation, whether through a bulk mixed matrix membranes, or as thin film composites (TFCs), the comparison is still instructive. This is effectively illustrated in modelling our observed results below, where we illustrate that the permeability and selectivity of the surface-modified PIM-1 can be predicted through a multi-layered model of varied intrinsic gas permeability so that the apparent ‘bulk’ values surpass the empirical upper-bound limitation of a homogeneous material, as shown in Figs 3e and 4 . The observed trends in selectivity and permeability as a function of ultraviolet irradiation time can be understood given that the exponentially decaying ultraviolet field generates a concentration gradient of ozone within the surface layer of the polymer. Making the broad assumption that ozone (and singlet oxygen) is responsible for the collapse of the PIM-1 framework, and hence the increase in local density and decrease in local permeability allows a determination of the overall and intrinsic permeability and selectivity of the membranes for different ultraviolet dosages. One such model calculation is given in Fig 3e, making a further assumption of a first-order oxidative chain scission reaction ( Supplementary Fig. S11 and Supplementary Note 1 ). An encouraging result of this model is the step-like depth-dependent permeability front that moves into the thin film over prolonged ultraviolet exposure time (as shown in Fig. 3f ) over similar time and length scales to the observed skin-layer structures. The model also allows prediction of overall permeability and selectivity of other important gas pairs, as shown in Fig. 4 . More details of this model will be provided in a future publication. However, it captures the essence of the observed structural changes but does not take into account the additional time-dependent effect of structural collapse on the diffusion of ozone in the polymer matrix. This explains why the model predicts a continued thickening of the skin layer into the bulk of the membrane ( Fig. 3f ) whereas in fact this slows down experimentally as the network above it collapses. In this study, the key contribution to the observed enhanced material properties arise from the role of ultraviolet-induced, internally generated oxidant in producing a dense selective surface skin to a high-permeability and porous material. The resulting asymmetric membrane geometry is analogous to TFC membranes. Nevertheless, from a chemical reaction viewpoint, the kinetics of photo-oxidation in PIM-1 could be tuned, that is, by controlling the intensity of ultraviolet irradiation, exposure time and oxygen concentration [O 2 ] within the polymer matrix. These parameters determine the concentration of intermediate species of ozone [O 3 ], singlet oxygen [O] and radicals within the polymer matrix. Therefore, it might be possible to scale-down the asymmetric pore structure on TFC membranes, to achieve higher selectivity while maintaining high permeance. As a rapid and simple processing technique, this implied modification of PIM-1 can be applied to various geometries of separation unit (for example, flat-sheet, spiral wound or hollow fibre configurations). Though the system has immediate application in dry gas atmosphere, the instability to condensable polar vapours solvents may initially limit its use in some industrial gas processing systems. For example, the membranes recovered the high permeability and low selectivity of fresh PIM-1 membranes after the ultraviolet/ozone-modified membrane had been immersed in polar solvents. This accelerated solvent test suggests that further post-treatment of the ultraviolet-modified surface is required to extend the applicability and endurance of the material. However, photo-oxidation introduces carbonyl and hydroxyl groups that can be used to stabilize the modified layer (for example, decarboxylation-induced crosslinking [36] , or thermal rearrangement [6] ). Conversely, with a strong resonance to techniques used in photolithography, the ultraviolet-generated rapid structural phase change should also make the material amenable to wet- and dry-etch photoresist and pattern development techniques. As a simple demonstration, PIM-1 films were exposed to ultraviolet light through a rudimentary edge-mask. A relatively clean, but unoptimized, topographical step profile was obtained after wet etching of the film with DMF ( Fig. 5 ). 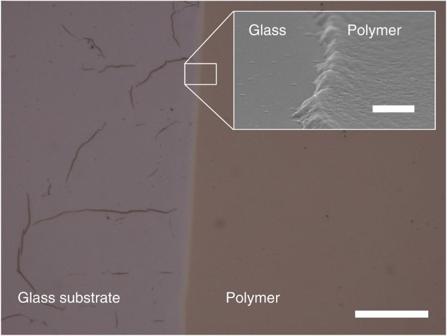Figure 5: Photoresist development. Optical microscopy image and SEM image (inset) of PIM-1 polymer thin film exposed to ultraviolet irradiation and wet etching with polar solvent. The PIM-1 polymer film (initial thickness of 300 nm) was exposed to ultraviolet irradiation in air for 10 min with the right half of the film protected by an overlying cleaved silicon wafer used as a basic mask; followed with wet etching in a polar solvent, DMF, the ultraviolet-exposed area was dissolved away in DMF as indicated by the interface shown in the inset SEM image. Scale bar, 100 μm (in optical image); 500 nm (in inset SEM). Figure 5: Photoresist development. Optical microscopy image and SEM image (inset) of PIM-1 polymer thin film exposed to ultraviolet irradiation and wet etching with polar solvent. The PIM-1 polymer film (initial thickness of 300 nm) was exposed to ultraviolet irradiation in air for 10 min with the right half of the film protected by an overlying cleaved silicon wafer used as a basic mask; followed with wet etching in a polar solvent, DMF, the ultraviolet-exposed area was dissolved away in DMF as indicated by the interface shown in the inset SEM image. Scale bar, 100 μm (in optical image); 500 nm (in inset SEM). Full size image A previous patent by the UOP company found that ultraviolet irradiation of PIM-1 polymer resulted in higher selectivity and compromised permeability and attributed this performance, without any scientific proof, to ultraviolet crosslinking of PIM-1 [47] . During the writing of this paper, Chung and co-workers reported similar phenomenon of PIM-1 polymer membranes sandwiched between quartz plates and exposed to ultraviolet irradiation; they proposed a rearrangement mechanism at the spiro centre [48] . There are no significant differences in the measured gas permeability reported in such work and this paper. However, the attribution of the performance to crosslinking (in the UOP patent) or chain rearrangement by Chung and co-workers is clearly in error. Here, we proposed a photo-oxidative surface modification mechanism based on the evidence of our physical and chemical characterizations. Specifically, we observed the evident loss of PIM-1 molecular weight upon ultraviolet irradiation (in air or quartz-sandwiched samples), the limited ultraviolet transmission within the polymer and formation of surface-densified layers. These observations deny the possibility of a bulk material transformation. In ruling out these other explanations, and by revealing the true physical transformation at work, we can invoke a simple reaction-controlled model of a surface-limited densification of the material. As seen by Figs 3d and 4 , the robustness of such a model is reinforced through its good predictions of apparent permeability in ultraviolet-transformed PIM-1 over a wide range of industrially important gas pairs. In summary, photo-oxidation can be a simple and powerful method to enhance the gas-separation performance of high free-volume polymeric molecular sieve membranes. These materials, and indeed other microporous materials, have an intrinsically greater potential for structural collapse than conventional dense polymers. The tight surface attenuation, due in part to the strong photo-absorbance in PIM-1, allows the generation of a sharp near-surface structural phase transition within the first few hundred nanometres of the material in an eminently tuneable fashion. Such controlled surface modification should be available through other analogous chemistry and can be used beyond the discussed separation application, for example, in microfabrication and coating technologies. Synthesis of polymer The PIM-1 polymer was synthesized following the method described by Budd and McKeown [11] , and an optimized recipe by Guiver and co-workers [49] . A one-step polycondensation via a double aromatic nucleophilic substitution from purified monomers, 5,5′,6,6′-tetrahydroxy-3,3,3′,3′-tetramethyl-1,1′-spirobisindane (TTSBI, 10.213 g, 30 mmol, Alfa Aesar) and 2,3,5,6-tetrafluoroterephthalonitrile (TFTPN, 6.003 g, 30 mmol, Matrix Scientific), was performed in the presence of K 2 CO 3 (8.292 g, 60 mmol, Aldrich) in anhydrous DMF (200 ml, Alfa Aesar). After the mixture has been stirred at 65 °C for about 40 h, the polymer was purified by dissolving in chloroform and reprecipitation from methanol, filtered and dried in vacuum oven at 110 °C for overnight. The molecular weight was determined from GPC, giving an average molecular weight of M n =100,000 Da and a polydispersity (PDI) of 1.8. Preparation of membrane Dense membranes were prepared by solution casting of filtered PIM-1 solution in chloroform on clean glass substrate, with solvent slow evaporated and removed. Thin films were prepared by spin coating or dip coating with diluted PIM-1 solution in chloroform. Photo-oxidation The membranes were exposed to ultraviolet irradiation ( λ =254 nm, incident intensity of 8.0 mW cm −2 ) in a commercial ultraviolet box (UVP model CX-2000). The membranes were exposed in air for exposure time studies. Alternatively, we controlled the atmosphere of ultraviolet irradiation using a temperature-controlled, quartz-windowed, stainless steel reactor with constant flow (100 ml min −1 , STP) of different gases. Characterization SEM analysis of membranes (fractured in liquid nitrogen) was performed using a Hitachi S5500 microscope. The molecular weight was quantified by GPC calibrated with polystyrene standards. Fourier Transform infrared spectroscopy of PIM-1 thin films, dip coated on NaCl plates after exposure to ultraviolet irradiation, were measured with a NICOLET spectrometer (iS10, Thermo Scientific) in transmission mode. Density values of both as prepared PIM-1 membrane and ultraviolet/ozone-treated samples were measured using a Micromeritics Accupyc 1340 helium pycnometer. Thermal analyses were performed in a thermogravimetric analyser (TGA) Q600 (simultaneous TGA–DSC). Nitrogen adsorption–desorption measurements at 77 K and CO 2 sorption at 293 K were carried out using a Micromeritics ASAP 2020 instrument. Nanoindentation was performed at ambient temperature using an MTS NanoIndenter ® XP (MTS Corp., Eden Prairie, MN), equipped with the continuous stiffness measurement module. A three-sided pyramidal Berkovich tip was used to determine the Young’s modulus ( E ) and hardness ( H ). Molecular simulation For molecular modelling, energy minimization and molecular dynamics were performed with the Materials Studio software package (Version 4.3, Accelrys Inc., CA, USA). In one amorphous cell, four PIM-1 polymer chains with ten repeating units were constructed. To mimic the chain scission, 20 short chains containing two repeating units of PIM-1 with oxidized groups were constructed in another amorphous cell as well. Optical spectroscopy methods Ultraviolet–visible absorption spectra of PIM-1 thin film (~100 nm, as measured by SEM) were measured using a Hewlett Packard 8453 ultraviolet–Vis spectrometer, with an operating spectral range of 190–1,000 nm. Steady-state photoluminescence excitation measurements were taken on CARY Eclipse fluorescence spectrophotometer, at an excitation wavelength of 420 nm. Gas permeation methods Pure gas permeation tests were carried out at a feed pressure of 4 bar and at temperature of 22 °C, using a constant volume pressure increase apparatus described elsewhere [50] . Mixed gas permeation was performed in another apparatus using the constant flow method, with certified gas mixtures of CO 2 /N 2 (50/50 vol.%) and CO 2 /CH 4 (50/50 vol.%) at feed pressure up to 35 bar at 22 °C. The stagecut, defined by permeate flow rate to feed rate (1,500 ml min −1 ) was less than 1%. The gas compositions were analysed by a gas chromatograph (GC-2014, Shimadzu). How to cite this article: Song, Q. et al . Photo-oxidative enhancement of polymeric molecular sieve membranes. Nat. Commun. 4:1918 doi: 10.1038/ncomms2942 (2013).